A low-temperature method to produce highly reduced graphene oxide Chemical reduction of graphene oxide can be used to produce large quantities of reduced graphene oxide for potential application in electronics, optoelectronics, composite materials and energy-storage devices. Here we report a highly efficient one-pot reduction of graphene oxide using a sodium-ammonia solution as the reducing agent. The solvated electrons in sodium-ammonia solution can effectively facilitate the de-oxygenation of graphene oxide and the restoration of π-conjugation to produce reduced graphene oxide samples with an oxygen content of 5.6 wt%. Electrical characterization of single reduced graphene oxide flakes demonstrates a high hole mobility of 123 cm 2 Vs −1 . In addition, we show that the pre-formed graphene oxide thin film can be directly reduced to form reduced graphene oxide film with a combined low sheet resistance (~350 Ω per square with ~80% transmittance). Our study demonstrates a new, low-temperature solution processing approach to high-quality graphene materials with lowest sheet resistance and highest carrier mobility. Graphene, a single layer of carbon arranged in a honeycomb structure, has attracted intense interest because of its fascinating electronic, thermal and mechanical properties. Graphene is typically prepared through mechanical cleavage or chemical methods. In particular, chemical exfoliation of graphene oxide (GO) either by ultrasonic dispersion or rapid thermal expansion followed by chemical reduction provides a low-cost and scalable method to produce bulk quantities of graphene flakes (or more commonly referred as reduced GO (RGO)) for possible applications in various fields including transparent conductors and energy-storage devices [1] , [2] , [3] , [4] , [5] , [6] , [7] , [8] , [9] . To date, many reduction reagents, such as sodium hydride [10] , hydrogen sulphide [11] , hydrazine [12] , NaBH 4 (ref. 13 ), dimethylhydrazine [14] , hydroquinone [15] , the sequential use of NaBH 4 and H 2 SO 4 (ref. 16 ), and aluminium powder [17] , have been used to reduce GO to produce RGO in the solution phase. The reduction of GO by pure hydrazine in the solution phase is particularly interesting because it can produce RGO of relative high quality with relatively small oxygen content [18] . Direct reduction of GO film has also been reported by exposure to hydrazine vapour and/or annealing at high temperature [19] , [20] , [21] , [22] . However, these approaches often involve highly toxic chemicals, require long reduction time, or require high-temperature treatment that are incompatible with flexible plastic substrates, and produce RGO with a relatively high oxygen content (~>9%) to give rise to high sheet resistance [23] . Recently, hydriodic acid with acetic acid has been reported for efficient conversion of GO thin film into RGO thin film, [24] which, however took over a day to produce RGO with 7.2% oxygen and generated toxic iodine vapour. It is therefore highly desired to develop new chemical reduction methods that involve less- or non-toxic chemicals for fast mass production of high-quality RGO with low oxygen content. Here we report a new method for the mass production of high-quality RGO and RGO films using sodium-ammonia (Na-NH 3 ) system (in dry ice-acetone bath). We show that Na-NH 3 solution can be used to effectively reduce GO and restore graphene structure at low temperature within a few minutes to produce with a lowest oxygen content of 5.6 wt%, and highest carrier mobility of 123 cm 2 Vs −1 . With the low-temperature reduction process, we further show that high-quality film can be directly produced on flexible substrate with the lowest sheet resistance of all solution-processed graphene thin films (~350 Ω per square versus >1,000 Ω per square at transmittance of ~80% for other approaches) by directly immersing the GO films in the Na-NH 3 solution for several minutes. Compared with other reported routes, including hydrazine reduction or directly thermal annealing, our strategy offers significant advantages because it not only produces graphene with a very low number of remaining functional groups and high conductivity in much shorter time (minutes versus days) and at low processing temperature but also provides a more environment-friendly protocol, not including the highly toxic reagents such as hydrazine or dimethylhydrazine. Production of RGO powder from electronic solution reduction Metallic sodium can be dissolved in liquid ammonia to create a blue solution with strong reducibility due to the generation of ‘solvated electron e − [NH 3 ] n ’ [25] , [26] , [27] . Dissolution of the sodium metal in the liquid ammonia results in ionization of the metal to form a sodium cation and a solvated electron strongly associated with the solvent ammonia ( Fig. 1a ). The deep blue colour of sodium metal in liquid ammonia solutions arises from the presence of solvated electrons (a free electron in a deep blue solution, Fig. 1b ). 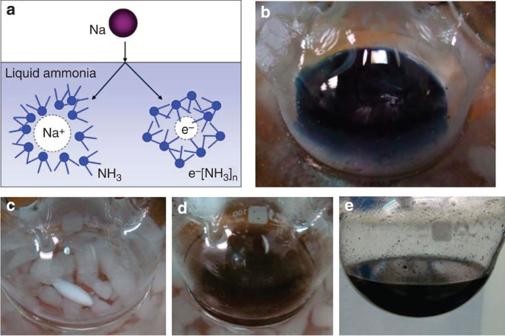Figure 1: Experimental procedures of the reduction of GO in Na-NH3system. (a) The generation of solvated electrons by dissolution of the sodium in liquid ammonia. (b) Several lump of sodium metal was then dissolved in anhydrous liquid ammonia. The deep blue colour is the colour of the solvated electrons. (c) Liquid ammonia was kept in dry ice-acetone bath. (d) GO powder was dispersed in liquid ammonia to show brown colour. (e) Black RGO solution was obtained after the reduction of GO with solvated electrons. Figure 1: Experimental procedures of the reduction of GO in Na-NH 3 system. ( a ) The generation of solvated electrons by dissolution of the sodium in liquid ammonia. ( b ) Several lump of sodium metal was then dissolved in anhydrous liquid ammonia. The deep blue colour is the colour of the solvated electrons. ( c ) Liquid ammonia was kept in dry ice-acetone bath. ( d ) GO powder was dispersed in liquid ammonia to show brown colour. ( e ) Black RGO solution was obtained after the reduction of GO with solvated electrons. Full size image The Na-NH 3 solution with the solvated electrons can function as a very potent electron source to effectively remove oxygen functionalities and restore the planar geometry of the GO sheets. In addition, with many intrinsic physical properties of liquid ammonia, such as polarity and hydrogen bonding, comparable to those of water, liquid ammonia can function as a good solvent to disperse GO. A photograph illustration of the typical procedure is shown in Fig. 1 . Dry GO powder was first dispersed in the liquid ammonia ( Fig. 1c ) and allowed to stir for 20 min to create stable dispersion of GO ( Fig. 1d ). Several lump of sodium metal was then dissolved in anhydrous liquid ammonia. After the reduction of GO with solvated-electron solution, a black RGO solution was obtained ( Fig. 1e ). The product was characterized systematically to confirm the production of single or few-layer RGO sheets. First, atomic force microscopy (AFM) was used to characterize the topographic height of sheets on mica substrate ( Fig. 2a ). A line scan of the height profile shows an average topographic height of ~0.91 nm, consistent with the typical height reported for single-layer graphene on mica substrate (~0.5–1.0 nm) [28] . Transmission electron microscopy (TEM) study was further used to investigate the morphology and crystalline structure of sheet. A representative TEM image of the as-produced RGO samples clearly shows the sheet-like nature of the material ( Fig. 2c ). Selected area electron diffraction shows that the sheets exhibit good crystallinity with the structure consistent with graphene (inset, Fig. 2c ) [29] , [30] . Scanning electron microscopy (SEM) images can be used to find large single sheets (>10 μm) of ( Fig. 2d ). 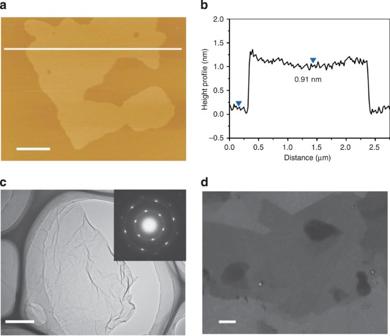Figure 2: Evidence for the dispersion of graphene sheets. (a,b) AFM image and its height profile of. (c) TEM image and selected area electron diffraction pattern ofnanosheet. (d) SEM image of largenanosheets. Such sheets are readily identified in SEM on silicon/SiO2substrates after spin coating from RGO dispersion. Figure 2: Evidence for the dispersion of graphene sheets. ( a , b ) AFM image and its height profile of . ( c ) TEM image and selected area electron diffraction pattern of nanosheet. ( d ) SEM image of large nanosheets. Such sheets are readily identified in SEM on silicon/SiO 2 substrates after spin coating from RGO dispersion. Full size image The powder X-ray diffraction was further used to characterize the bulk structure of the prepared ( Fig. 3a ). A typical broad peak near 10.21° ( d -spacing ~8.67 A) was observed for the GO powder. Compared with the parent GO, the peak of shows a obvious shift to higher 2 θ angles (25.04°; d -spacing ~3.56 A) and is narrower than that of highly RGO (~23°; d -spacing ~3.86 A) obtained previously [22] , suggesting that was well ordered with two-dimensional sheets with more thorough removal of surface functional groups. 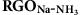Figure 3: Characterization ofpowder. (a) X-ray diffraction (XRD) patterns of graphite, GO andpowder. The 2θangles of the XRD peaks (d-spacing) of GO andshifted from 10.21° (d-spacing ~8.67 A) to 25.04° (d-spacing ~3.56 A) after reduction. (b) XPS spectra of graphite, GO and. (c) TGA thermograms for GO,and. (d) Raman spectra of GO,andpowder. Figure 3: Characterization of powder. ( a ) X-ray diffraction (XRD) patterns of graphite, GO and powder. The 2 θ angles of the XRD peaks ( d -spacing) of GO and shifted from 10.21° ( d -spacing ~8.67 A) to 25.04° ( d -spacing ~3.56 A) after reduction. ( b ) XPS spectra of graphite, GO and . ( c ) TGA thermograms for GO, and . ( d ) Raman spectra of GO, and powder. Full size image X-ray photoemission spectroscopy (XPS) was used to investigate the chemical structure and composition of the prepared powder samples. Figure 3b shows the C1s spectra of graphite, GO and powder samples. In general, the exhibits the similar XPS spectrum to that of the natural graphite ( Fig. 3b , Supplementary Figs S1 and S7 ), C=C bonds dominate, as shown by one single peak with small tails at the higher-binding energy region, confirming the good restoration of C=C bonds in the . In contrast, the original GO signal shows two separated peaks because of the high percentage of oxygen functionalities. Furthermore, we have obtained the atomic composition (wt%) of all the samples by XPS. Significantly, our sample shows a lowest oxygen percentage (5.62 wt%) and nitrogen percentage (0.86 wt%). Our products are quite distinct from all the other RGOs, such as a hydrazine reduction product (oxygen wt% 11.57%, nitrogen wt% 3.78%) [31] ( Supplementary Table S1 ). Raman spectroscopy provides a non-destructive method for characterizing graphene. Graphene typically exhibits three main Raman features, G-band, D-band and two-dimensional modes, each having different physical origins [32] . Raman spectra of GO and and powder are shown in Fig. 3d , recorded using 514 nm laser irradiations. The I D / I G ratio of did increase notably, indicating that the reduction process altered the structure of GO [32] , [33] . It is particularly important to note that the intensity of the two-dimensional peak of is much stronger than that of , suggesting a better graphitization in [18] . Thermogravimetric analysis (TGA) was used to further assess the level of reduction of the GO platelets. Figure 3c displays the TGA thermograms that show weight loss as a function of temperature for dried-down GO and (at a heating rate of 10 °C min −1 ) under a nitrogen atmosphere. The GO sample showed significant weight loss with an onset temperature at slightly >100 °C, which was attributed to the elimination of interlamellar water, followed by loss of oxygen from the GO platelets themselves at slightly higher temperatures. showed much higher thermal stability because of the more complete de-oxygenation and better graphitization with enhanced van der Waals forces between layers [34] , [35] , [36] . To probe the fundamental mechanism for the reduction of GO with solvated electrons, we have carried out detailed Fourier transform infrared spectroscopy (FTIR) study to monitor the evolution of the functional groups in GO during the reduction process. Importantly, FTIR spectra clearly show the progressive removal of the oxygen groups by solvated electrons ( Supplementary Figs S2 and S3 ). As the GO films are reduced by solvated electrons, peaks for all oxygen functional groups are significantly reduced or entirely removed ( Supplementary Fig. S2 ). In general, the oxygen-containing groups can readily accept solvated electrons to cleave carbon-oxygen bond and form carbon radical or radical anion on the plane of GO [25] , [26] ( Supplementary Fig. S4 ). The solvated electrons and the partially delocalized π-conjugation in the GO plane could stabilize the carbon radicals [26] , [27] to facilitate the formation of π-bond and restoration of the π-conjugation in graphene resulting in high-quality RGO ( Supplementary Fig. S5 ). Fabrication and characterization of the RGO film RGO films were usually obtained on a membrane filter by vacuum filtration of as-reduced RGO dispersions [36] . However, the dispersion of RGO sheets in solution is usually much more difficult than GO. Ruoff and co-workers have recently demonstrated that strong GO paper can be prepared using a similar filtration strategy [36] . To make the resulting GO film conducting, an additional reduction step was needed by either exposing to hydrazine vapour and/or annealing in inert conditions. However, the hydrazine vapour alone is not sufficient to achieve optimum reduction [19] , and annealing alone requires relatively high temperatures. Importantly, with Na-NH 3 as the reduction agent in our approach, GO film can be readily converted into uniform RGO film within just several minute at low temperature ( Fig. 4a–c and Supplementary Fig. S6 ). Here the solvated electrons allow highly efficient reduction and the rapid de-oxygenation at mild conditions to obtain the best recovery of the graphene-conjugated structure. This low-temperature solution reduction process is especially important for the graphene-based flexible transparent conductive electrodes that require low processing temperature. 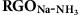Figure 4: Flexiblethin films with GO reduced in the Na-NH3solution. (a) The blue Na-NH3solution. (b) GO/PVDF film. (c)/PVDF film produced by directly dipping in Na-NH3solution for 1 min. (d) SEM image of the surface of thefilm. Scale bar, 1 μm. (e) Flexible GO thin film on a PET substrate. (f) Flexiblethin film on a PET substrate. (g) Water contact angles: (1) GO (65.3°),/PVDF film dipping in Na-NH3solution at (2)t=1 min (87.6°), (3)t=5 min (93.2°) and (4)t=10 min (99.7°). (h) Sheet resistance of the RGO films by dipping in the Na-NH3solution at different time. (i) Raman spectra of GO film and RGO films by dipping in the Na-NH3solution at different time. Figure 4: Flexible thin films with GO reduced in the Na-NH 3 solution. ( a ) The blue Na-NH 3 solution. ( b ) GO/PVDF film. ( c ) /PVDF film produced by directly dipping in Na-NH 3 solution for 1 min. ( d ) SEM image of the surface of the film. Scale bar, 1 μm. ( e ) Flexible GO thin film on a PET substrate. ( f ) Flexible thin film on a PET substrate. ( g ) Water contact angles: (1) GO (65.3°), /PVDF film dipping in Na-NH 3 solution at (2) t =1 min (87.6°), (3) t =5 min (93.2°) and (4) t =10 min (99.7°). ( h ) Sheet resistance of the RGO films by dipping in the Na-NH 3 solution at different time. ( i ) Raman spectra of GO film and RGO films by dipping in the Na-NH 3 solution at different time. Full size image To accomplish this, GO thin film or paper was first prepared by vacuum filtration of a GO dispersion through a polyvinylidene fluoride (PVDF) (or alumina) membrane ( Fig. 4b ). Next, the GO/PVDF film was directly dipped into the deep blue Na-NH 3 solution ( Fig. 4a ). The brownish GO/PVDF film quickly turned to black within less than 1 min in the Na-NH 3 solution. The black RGO film was taken out, washed with de-ionized water and dried at room temperature ( Fig. 4c ). The SEM image of the surface of the film is revealed in Fig. 4d . AFM studies show that RGO film exhibits a similar kinked and wrinkled surface morphology to that of GO film before reduction ( Supplementary Fig. S8 ), suggesting that the reduction does not significantly alter the physical appearance of the GO films. The resulting GO and RGO film can be further peeled off the membrane and transferred onto a polyethylene terephthalate (PET) film ( Fig. 4e ) for electronic applications. The degree of reduction of the films was further assessed by their hydrophobicity. Figure 4g shows the wettability of the GO and obtained with different immersion time. The water contact angles of the GO, thin films for 1, 5 and 10 min reduction were 65.3°, 87.6°, 93.2° and 99.7°, respectively ( Fig. 4g ). Clearly, the surface had the higher hydrophobicity, indicating a high degree of reduction and more complete removal of oxygen contents [24] . Sheet resistance of the reduced films is another important parameter to evaluate how the π -conjugated system has been restored in the RGO film. Figure 4h shows that the sheet resistances decreased substantially with the increasing reduction time and quickly approached a steady value within 5 min. Significantly, a low sheet resistance ~350 Ω per square is achieved in an ultra-thin film of RGO with ~80% transparency, which represents the lowest sheet resistance achieved in solution-processed RGO film to date [19] , [24] ( Supplementary Figs S9 and S10 , Supplementary Table S2 ). The low sheet resistance observed in our thin film is consistent with the highest degree of de-oxygenation and graphitization. To further verify the high quality of the RGO sheets, we have also fabricated field-effect transistors based on individual RGO flakes and performed the corresponding electrical measurements ( Supplementary Fig. S11 ). These studies show that a single-layer RGO flake exhibits a hole mobility of 123 cm 2 V −1 s −1 , which represents the highest mobility value achieved solution-processed RGO materials to date ( Supplementary Table S3 ), further demonstrating the unusually high quality of the RGO sample obtained with our approach. The restoration of the conjugated C=C bonds during the chemical reduction of GO to RGO film was observed in their Raman spectra. A monotonic increase of the D/G intensity ratio for the films with increasing reduction time was observed ( Fig. 4i ). The RGO films show much narrower Raman peaks than the GO film. Although a prominent D peak is typically an indication of disorder in the Raman of peeled graphene, our observations are consistent with previous reports of RGO materials [28] . A greater ratio of the Raman D/G intensity of the films compared with the GO film indicates an increase in the number of smaller sp 2 domains [33] , [34] . We have demonstrated that thin films can be readily formed by controlled chemical conversion of GO films in the Na-NH 3 solution, which is a clean, safe and ultrafast method. The resulting paper could find use in many fields, including membranes, anisotropic conductors and supercapacitors. The successful formation of graphene film from GO film and GO coating by directly dipping in the Na-NH 3 solution holds great potential in many applications, such as sensors and neuroprosthetic devices, and can lead to the development of a new generation of antistatic coatings that combine electrical conductivity with transparency, excellent thermal and chemical stability, water resistance and low production cost. RGO-based supercapacitors To demonstrate the multifunctionality of the RGO film in a variety of large-scale applications, we have explored the RGO films for supercapacitors. Graphene materials have recently been used in supercapacitor [37] , [38] devices to replace conventional carbon electrodes and have shown very good performance. 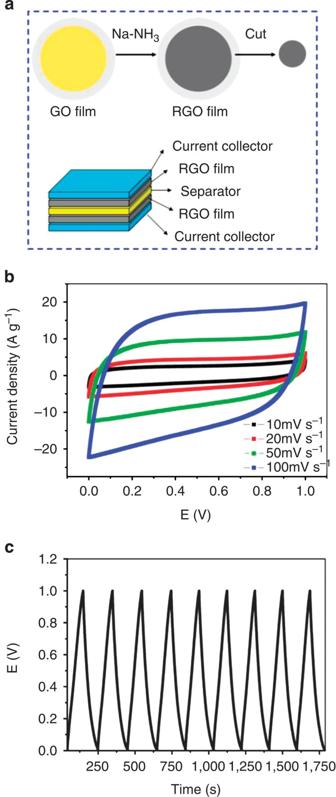Figure 5: RGO film-based supercapacitor device. (a) Schematic diagram of RGO film-based supercapacitor device. (b) Cyclic voltammograms of RGO film-based supercapacitor obtained at various scan rates. (c) Charge–discharge behaviour of RGO film-based supercapacitor performed at 1 A g−1. The slope of the discharge curve was used to calculate the value of specific capacitance. Figure 5a schematically illustrates the process flow to use our RGO film for the flexible supercapacitor electrodes. To achieve optimum capacitance, it is important to maintain a high surface area in the RGO film. To this end, the direct reduction of pre-formed GO film into RGO film can present a unique advantage. In general, because of electrostatic repulsion between GO flakes (GO usually possesses a large number of negative charges due to carboxylic groups), and random wrinkling, folding in the film-formation process, GO film is usually more porous than the film processed directly from RGO (with strong flake-to-flake pi–pi stack interaction). After the formation of GO film, all the GO flakes are locked in place and do not have much freedom to move during the reduction process. Therefore, a direct reduction of GO film can minimize the re-stack of the graphene sheets to allow the formation of RGO film with much better porosity ( Supplementary Fig. S12 , specific surface area of 648 m 2 g −1 ) than that processed directly from RGO solution (specific surface area of 330 m 2 g −1 ). In addition, to further retain a high surface area, we have directly used the freshly reduced wet RGO films as the capacitor electrodes without drying the film, which can prevent capillary drying effect and the re-stack of the graphene sheets [38] . Figure 5: RGO film-based supercapacitor device. ( a ) Schematic diagram of RGO film-based supercapacitor device. ( b ) Cyclic voltammograms of RGO film-based supercapacitor obtained at various scan rates. ( c ) Charge–discharge behaviour of RGO film-based supercapacitor performed at 1 A g −1 . The slope of the discharge curve was used to calculate the value of specific capacitance. Full size image The performance of our supercapacitors was characterized through cyclic voltammetry ( Fig. 5b ) and galvanostatic charge–discharge measurements ( Fig. 5c ). The measurements demonstrate that our supercapacitor possess a specific capacitance as high as 263 F g −1 (see Supplementary Method ). Without the use of any binder or specially prepared current collector, our supercapacitors represent a significant improvement over previously reported carbon nanotube-based supercapacitors (51 F g −1 ) [39] and are substantially better than those obtained with less reduced (99 F g −1 ) [37] , and compares well with the recently reported laser reduced GO supercapacitors [40] . In conclusion, by using Na-NH 3 treatment with active solvated electrons as the highly reductive agent, we have devised a simple and effective method to restore graphene structure with the lowest oxygen content (5.6%) and the highest carrier mobility (123 cm 2 Vs −1 ) of all solution-reduction process. We have also shown that this approach can be used to directly reduce the pre-formed GO thin film into RGO film with a combined low sheet resistance (~350 Ω per square) and good optical transparency (~80% transmittance). Furthermore, the simplicity and low-temperature process of this method demonstrates the possibility of mass-production RGO and RGO thin film with high conductivity on plastic substrates. Our approach thus offers a great deal of flexibility in the creation of graphene film and novel graphene-based materials and devices. This cheap and simple procedure is of great significance not only for future nanoelectronics but also for large-scale applications such as transparent flexible electronics, antistatic coatings, electrochemical devices and conductive nanocomposites and so on. Preparation of GO GO was prepared from natural graphite powder (Bay Carbon; SP-1 graphite) using the modified Hummers method [22] , [41] . Preparation of and In a typical procedure, 500 mg of GO was dispersed in 100 ml of liquid NH 3 . This dispersion was stirred for 20 min until it became clear. Na (800 mg, cutting into small) was then added and the mixture was stored at dry ice-acetone bath for 30 min with constant stirring. We then removed the ice-acetone bath and let the ammonia volatize to remove it. The product was isolated by filtration, washed with distilled water and ethanol and then vacuum dried overnight at room temperature to yield RGO. The powder was reduced from GO with hydrazine hydrate using the Wallace method [32] . Fabrication of GO and RGO thin films A dilute GO suspension was vacuum filtered using a mixed cellulose ester membrane with 20 nm pores (Millipore). The GO film was allowed to dry and adhered to the substrate at room temperature overnight under a 5.0-kg weight. The weight was removed and the membrane was dissolved in acetone to leave the GO thin film on the substrate. The GO film was then rinsed with methanol and carefully transferred onto a PET film. A dilute GO suspension was vacuum filtered using a PVDF membrane with 20 nm pores (Millipore). The GO/PVDF film was dipped into a Na-NH 3 solution for several minutes. Subsequently, the RGO/PVDF film was rinsed with saturated sodium bicarbonate, water and methanol, and dried at room temperature. The colour of the RGO/PVDF film changed from pale brown to black. RGO/PVDF film can be peeled off the membrane and transferred onto a PET substrate. We also used the alumina membrane (40–70 nm) to transfer the RGO film onto a PET substrate. Characterization The AFM measurements were performed with a SPI 4000 system in tapping mode. The samples were deposited from ethanol suspension onto freshly cleaved mica substrates, dried by evaporation, and the measurements were performed in air at ambient temperature and pressure. TEM and high-resolution TEM and electron diffraction images were obtained using a JEM-1200EX. The TEM samples were prepared by drying a droplet of the graphene suspension on holey carbon grids. SEM imaging was performed using a JSM 7401F. The SEM samples were prepared by depositing materials onto a silicon substrate by drop drying. The FTIR spectrum (800–4,000 cm −1 ) was measured using a Perkin Elmer FTIR spectrometer with pure KBr as the background. After purification by filtration and repeated washing, the GO and RGO samples were collected and ground with KBr. The mixture was dried and compressed into a transparent tablet for measurement. We prepared the RGO samples at different reduction stages for the detailed FTIR studies by controlling the reduction time in the Na-NH 3 solution. XPS measurements were conducted with an ESCALab220i-XL electron spectrometer from VG Scientific using 300 W Al (Kα) radiation. The base pressure was about 3 × 10 −9 mbar. The binding energies were referenced to the C1s line at 284.8 eV from adventitious carbon. Samples were prepared by filtration and repeated washing. The graphite powder was used for XPS measurement without any treatment. Raman spectroscopy was performed on a Renishaw RM2000 microscopic confocal Raman spectrometer (Gloucestershire, UK) using green (514 nm) laser excitation. Scans were taken on an extended range (1,000–3,500 cm −1 ). A sample was sonicated in ethanol and drops applied to a glass slide for observation. Raman spectra of solid samples were taken by depositing the graphite on a glass slide. X-ray diffraction data were collected on a Bruker D8-Advance using Cu-Kα radiation ( λ =1.5418 Å). The thermal properties of the graphene platelets were characterized by TGA (Polymer Laboratories; TGA 1000 plus). All RGO sample measurements were taken at a nitrogen gas flow rate of 40 ml min −1 over a temperature range of room temperature to 800 °C with a ramp rate of 10 °C min −1 . The contact angles were measured using a SEO Phoenix 300 microscope at five different points. Conductivity measurements of films prepared by vacuum filtration were carried out on a Jandel RM3 Test Unit using a four-probe conductivity test metre at room temperature. The electrochemical tests for RGO-based supercapacitor was carried out in a standard three-electrode system controlled with a Princeton Versa Stat 3 electrochemical working station ( Supplementary Fig. S13 ). How to cite this article: Feng, H. et al . A low-temperature method to produce highly reduced graphene oxide. Nat. Commun. 4:1539 doi: 10.1038/ncomms2555 (2013).